Geometry analysis and systematic synthesis of highly porous isoreticular frameworks with a unique topology Porous coordination polymers are well known for their easily tailored framework structures and corresponding properties. Although systematic modulations of pore sizes of binary prototypes have gained great success, simultaneous adjustment of both pore size and shape of ternary prototypes remains unexplored, owing to the difficulty in controlling the self-assembly of multiple molecular building blocks. Here we show that simple geometry analysis can be used to estimate the influence of the linker lengths and length ratios on the synthesis/construction difficulties and framework stabilities of a highly symmetric, ternary prototype composed of a typical trinuclear metal cluster and two types of bridging carboxylate ligands. As predicted, systematic syntheses with 5×5 ligand combinations produced 13 highly porous isoreticular frameworks, which show not only systematic adjustment of pore volumes (0.49–2.04 cm 3 g −1 ) and sizes (7.8–13.0 Å; 5.2–12.0 Å; 7.4–17.4 Å), but also anisotropic modulation of the pore shapes. Systematic modulation of the pore size and shape of porous materials, especially without changing the structural prototype (connectivity or topology), is a rational strategy to enhance or optimize adsorption and separation performances. Compared with conventional adsorbents, porous coordination polymers (PCPs) or metal-organic frameworks are unique because of their designable frameworks and adjustable pore metrics (size/shape/surface) [1] , [2] , [3] , [4] , [5] . For example, linear dicarboxylates (L 2 ) with different lengths and/or side groups have been incorporated into the pcu (lower-case, boldfaced three-letter notation for topological type) structure Zn 4 O(L 2 ) 3 , although interpenetration sometimes occurs [6] , [7] , [8] , [9] , [10] , [11] , [12] , [13] , [14] . Nevertheless, until now, only very few prototypes have been systematically modulated, including the [M 2 (L 4 )(L 1 ) 2 ] ( nbo net, L 4 =tetracarboxylate, L 1 =monodentate ligand) [15] , [16] , [17] , [18] , [19] , M 2 (L 6 ) 2/3 (L 1 ) 2 ( rht net, L 6 =hexacarboxylate) [18] , [20] , [21] , [22] , [23] , [24] , M 3 (μ 3 -O)(L 2 ) 3 (L 1 ) 3 ( acs net) [25] , [26] and so on [27] , [28] , [29] , [30] , [31] , [32] . In these binary prototypes composed of only one kind of node and one kind of linker, the linker length controls the pore size rather than the pore shape. Alternatively, modulation of the pore shape can be implemented by changing the length ratio of the two types of linkers in the ternary prototypes (that is, one kind of cluster and two kinds of ligands). However, for most ternary systems, changing the length ratio of two types of ligands usually gives rise to diverse topologies. For example, connecting the Zn 4 O(O 2 CR) 6 clusters by mixed dicarboxylates and tricarboxylates with different lengths produces PCPs with a general formula, Zn 4 O(L 2 )(L 3 ) 4/3 (L 3 =tricarboxylate), but different topologies such as muo , toz or ith-d [33] , [34] , [35] , [36] , [37] . Typical pillared-layer structures can change their pore heights by changing the pillar ligands, but their pore widths, determined by the layer structures, are generally unchangeable [38] , [39] , [40] , [41] . Although the jungle-gym-type framework Zn 2 (L 2 ) 2 (L 2N ) ( pcu net, L 2N =exobidentate ligand similar to 4,4′-bipyridine) seems promising, most reported examples possess only one-dimensional square-shaped channels, because interpenetration occurs when the bipyridyl-type ligand is lengthened [42] , [43] , [44] , [45] , [46] , [47] . In short, systematic modulation of both pore size and shape remains largely unexplored and requires an in-depth understanding of the construction principle from molecular building blocks to network prototypes. A recently reported porous metal carboxylate framework, [Ni II 2 Ni III (μ 3 -OH)(pba) 3 (ndc) 1.5 ] (MCF-19), constructed from the Ni 3 (μ 3 -OH)(O 2 CR) 6 (L 1 ) 3 clusters, pyridylbenzoates and naphthalenedicarboxylates with a 2:6:3 ratio, represents a novel ternary prototype, because it possesses not only an unprecedented, uninodal, nine-connected ncb topology, but also a unique hierarchical channel-cavity biporous system [48] , [49] . Although a combination of two kinds of long linkers with similar lengths has been suggested as the key point for such an inherently tensile network, how ligand lengths (including length ratio) control the pore size/shape or even the construction possibility is not straightforward. In this report, these issues are addressed by using a geometry analysis approach, which is confirmed by the successful prediction of the outcome for a large-scale systematic synthesis with 5×5 linker combinations. Detailed characterization of the new series of 13 highly porous isoreticular frameworks shows that ligand lengths have an important role in determining not only the pore size, pore volume and surface area, but also the pore shape, framework distortion/stability and gas sorption behavior. Reticular modelling and geometry analysis The ncb net (the maximum lattice symmetry is the space group I -43 m ) has one kind of vertex (V, 3 m symmetry, x = y = z =0.1875) and two kinds of edges (E 1 and E 2 with m and mm 2 symmetries, respectively). Note that in an ideal ncb net, E 1 and E 2 have equal lengths (that is, E 1 / E 2 =1) [50] . The overall connectivity can be simplified as a body-centred cubic array ( bcu topology) of triakis tetrahedra; that is, a central regular tetrahedron (4V+6E 2 ) capped by four regular trigonal pyramids (4V+3E 1 +3E 2 , regular tetrahedral shape when E 1 / E 2 =1), connected in a cusp-to-umbilicus fashion ( Fig. 1a ). 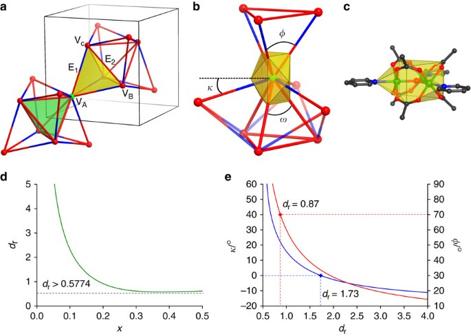Figure 1: Geometry analysis of the ncb net. (a) Perspective view of a fragment (only the cubic unit cell and two triakis tetrahedra, one at the centre and the other at the corner of the unit cell, are shown for clarity) of thencbnet composed of one kind of vertex (aka node) and two kinds of edges (red-blue and red sticks for E1and E2, respectively) at its maximum symmetry ofI-43m(black lines for unit cell). The ratiodrbetween the lengths of E1and E2can be calculated from the fractional coordinates or vertexes VA(x,y,z), VB(−y+0.5,x+0.5, −z+0.5), and VC(y+0.5, −x+0.5, −z+0.5) according to the crystal symmetry. (b) The node geometry can be described by three parameters (κ, φ, ω), two of which (κ, φ) are dependent ondr. The node geometry in the idealncbnet obviously deviates (dr=1, κ=15.7°) from the ideal tricapped trigonal-prismatic geometry. (c) Perspective view of a common nine-connected trinuclear M3(μ3-O)(O2CR)6(L1)3cluster showing the tricapped trigonal-prismatic geometry. (d) Mathematical relation ofdrand the node positionx(x=y=z). (e) Mathematical relation of the node geometry (κ, φ) anddr. Figure 1: Geometry analysis of the ncb net. ( a ) Perspective view of a fragment (only the cubic unit cell and two triakis tetrahedra, one at the centre and the other at the corner of the unit cell, are shown for clarity) of the ncb net composed of one kind of vertex (aka node) and two kinds of edges (red-blue and red sticks for E 1 and E 2 , respectively) at its maximum symmetry of I -43 m (black lines for unit cell). The ratio d r between the lengths of E 1 and E 2 can be calculated from the fractional coordinates or vertexes V A ( x , y , z ), V B (− y+ 0.5, x +0.5, − z +0.5), and V C ( y +0.5, − x +0.5, − z +0.5) according to the crystal symmetry. ( b ) The node geometry can be described by three parameters ( κ, φ, ω ), two of which ( κ, φ ) are dependent on d r . The node geometry in the ideal ncb net obviously deviates ( d r =1, κ=15.7°) from the ideal tricapped trigonal-prismatic geometry. ( c ) Perspective view of a common nine-connected trinuclear M 3 (μ 3 -O)(O 2 CR) 6 (L 1 ) 3 cluster showing the tricapped trigonal-prismatic geometry. ( d ) Mathematical relation of d r and the node position x ( x=y=z) . ( e ) Mathematical relation of the node geometry ( κ, φ ) and d r . Full size image The nine-connected node in the idealized ncb exhibits a distorted tricapped trigonal-prismatic geometry (point group symmetry C 3 v ; Fig. 1b ), which obviously deviates from the regular ones ( D 3 h ) and the most similar secondary building units (SBUs; Fig. 1c , see discussion below) on the three capped sites. Nevertheless, the connectivity and crystal symmetry can be retained when moving the vertexes along the space diagonals of the unit cell ( x = y = z , 0< x <0.5). But at the same time, the relative edge length ( d r = E 1 / E 2 ) and the node geometry will be altered, which is realistic because the lengths of pyridylcarboxylate and dicarboxylate are generally unequal. Using simple geometry calculations ( Supplementary Fig. S1 ; Supplementary Methods ), we deduced the relation between the node position and the relative edge length ( Fig. 1d ; Supplementary Fig. S2 ), in which a minimum of d r =0.5774 at x =0.375 represents the fusion of triakis tetrahedra into tetrahedra ( Supplementary Fig. S3 ). Owing to their regular tricapped trigonal-prismatic geometry, the trinuclear M 3 (μ 3 -O)(O 2 CR) 6 (L 1 ) 3 clusters ( D 3 h ) are the most appropriate candidates for the nine-connected node (using a ditopic ligand to function as two monodentate ligands L 1 ), although distortion must occur when a real ncb network is constructed. To evaluate the difference in geometry between the node and the SBU, three parameters are required to describe the node geometry ( Fig. 1e ); that is, κ for the deviation angle of the E 1 edge from the ideal capped position, φ for the angle between two adjacent E 1 edges, and ω for the angle between two adjacent E 2 edges. Obviously, κ and φ are dependent on d r , but ω is a constant (60°), as it is a part of the central regular tetrahedron. It can easily be identified from the diagram that the ideal ncb net ( x =0.1875, d r =1) possesses a geometry with φ =60° and κ =15.7°, implying that connecting the M 3 (μ 3 -O)(O 2 CR) 6 (L 1 ) 3 clusters by ligands with equal lengths may not be the best construction strategy. Although κ can approach zero to match the SBU geometry, φ will be very small at the same time, which may result in a large steric hindrance between the adjacent carboxylates. For example, when κ =0° at d r =1.73, the corresponding φ =33.5° is far smaller than the angles between the nearest carboxylate groups in common discrete M 3 (μ 3 -O)(O 2 CR) 6 (L 1 ) 3 clusters (ca. 70°), whereas when φ approaches the ideal value of 70° at d r =0.87, κ =23.2° causes a large distortion on the pyridyl binding sites. In other words, not only κ but also φ determine the inner tension and/or the possibility to construct real ncb networks. Therefore, a reasonable d r value should be close to 0.87–1.73 for a balance between κ and φ . Considering that the included angle between carboxylates in common six-connected M 3 (μ 3 -O)(O 2 CR) 6 (L 1 ) 3 clusters can be changed in a certain range (28~90°) to give dynamic breathing frameworks ( acs net) [51] , adjusting φ might be easier than changing κ , suggesting that an optimum d r should be closer to 1.73 rather than 0.87. In addition, as ω (60°) is also smaller than the angle between the nearest carboxylate groups in the SBUs (70°), the dicarboxylate ligand should have enough flexibility (or length) to compensate for the deviation. Combinatorial syntheses To verify the above analyses, a cross 5×5 ligand combination of (quasi-)linear pyridylcarboxylates (isonicotinate (ina − ), ( E )-3(pyridine-4-yl)acrylate (pyac − ), 4-(pyridine-4-yl)benzoate (pba − ), ( E )-4-(2-(pyridine-4yl)vinyl)benzoate (pvba − ), 4′-(pyridine-4-yl)biphenyl-5-carboxylate (pbpa − )) and dicarboxylates (benzene-1,4-dicarboxylate (bdc 2– ), naphthalene-2,6-dicarboxylate (ndc 2– ), biphenyl-4,4′-dicarboxylate (bpdc 2– ), ( E )-4,4′-(ethene-1,2-diyl)dibenzoate (edba 2– ), p -terphenyl-4,4″-dicarboxylate (tpdc 2– )) with successively increasing lengths (ca. 2.2 Å per step, see Supplementary Table S1 ) was employed to construct the targeted ncb network. Notably, ina − is the shortest pyridylcarboxylate, and bdc 2– is the shortest known dicarboxylate that can connect the M 3 (μ 3 -O)(O 2 CR) 6 (L 1 ) 3 SBUs into a regular tetrahedral cage. To calculate the hypothetic node geometries, not only the ligand lengths but also the volume of the SBU (distances between donor atoms and the center of the SBU, which are 3.2 Å for the carboxylate and 4.0 Å for the pyridyl) was considered. Although the calculations showed that some combinations exceeded the optimum interval of d r ( Supplementary Table S1 ), all 5×5 ligand combinations were tried in the synthetic experiments, and all the solid products obtained were subjected to powder and/or single-crystal X-ray diffraction analyses ( Supplementary Figs S4–S29 ; Supplementary Tables S2 and S3 ). So far, 13 isoreticular open frameworks (denoted as Ia , IIa , IIb , IIIa , IIIb , IIIc , IVa , IVb , IVc , Va , Vb , Vc and Vd ) with the expected ncb topology and the general formula [Ni II 2 Ni III (μ 3 -OH)(L P ) 3 (L 2 ) 1.5 ] (L P =pyridylcarboxylate) have been successfully isolated from the 15 ligand combinations with 0.87< d r <1.73 ( Supplementary Figs S30–S32 ). For ligand combinations with d r <0.87, only amorphous solids or other undesired products have been found under the various tested synthetic conditions (different solvents, temperatures, additives and so on have been tried). Also, attempts to synthesize several structures with d r close to 0.87 and/or 1.73 still resulted in low yields and poor reproducibility ( Supplementary Fig. S29 ; Supplementary Table S2 ). These results indicate that d r can be used to predict the difficulty in the synthesis of ncb -type frameworks. As shown in Supplementary Table S1 , the ligand combination with d r >1.73 requires an extremely long pyridylcarboxylate ligand, such a ligand is beyond the range of our examination. Crystal structures All isoreticular frameworks obtained are basically isostructural ( Fig. 2a ; Supplementary Figs S4–S28 ; Supplementary Table S3 ). The planar Ni 3 (μ 3 -OH) core units are encapsulated by six carboxylate groups (from the three dicarboxylates and three pyridylcarboxylates) and three pyridyl groups (from other three pyridylcarboxylates), forming nine-connected tricapped trigonal-prismatic SBUs ( Supplementary Table S4 ). As defined by the tiling of the ncb topology (1[3 4 ]+4[3 4 ]+3[3 4 .4 4 ]), all compounds obtained possess tetrahedral, trigonal-pyramidal and quasi-bisdisphenoidal cavities (denoted as cA, cB and cC, respectively) in a 1:4:3 ratio. Each cA connects with four cBs through small apertures (the aperture between cA and cB, denoted as aAB) to form a triakis tetrahedral cage, which is arranged in a bcu array, but is isolated from each other. Each cC connects to four neighbors through large apertures (aCC) to form a three-dimensional intersecting nbo channel (dual of bcu ). Finally, the isolated bcu cavities connect to the nbo channel through small apertures between cB and cC (aBC), furnishing a hierarchical channel-cavity biporous system ( Fig. 2b ). 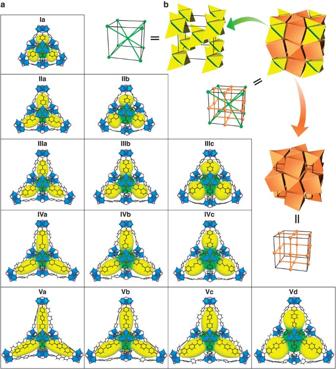Figure 2: X-ray single-crystal structures and topology of pore systems. (a) Perspective views of the triakis tetrahedral building units with the pore surface of the embedded cA (green) and cB (yellow) cavities of the obtained isoreticular frameworks listed in the same order as inSupplementary Table S1. (b) The pore system defined by the isoreticularncbframeworks is an interpenetrated network between abcuarray of isolated triakis tetrahedra composed of one tetrahedron (cA, green) with four trigonal pyramids (cB, yellow) and annboarray of quasi-bisdisphenoids (cC, orange). Note that the topologiesncb,bcuandnboall possess the cubic symmetry (black lines represent the unit cell). Figure 2: X-ray single-crystal structures and topology of pore systems. ( a ) Perspective views of the triakis tetrahedral building units with the pore surface of the embedded cA (green) and cB (yellow) cavities of the obtained isoreticular frameworks listed in the same order as in Supplementary Table S1 . ( b ) The pore system defined by the isoreticular ncb frameworks is an interpenetrated network between a bcu array of isolated triakis tetrahedra composed of one tetrahedron (cA, green) with four trigonal pyramids (cB, yellow) and an nbo array of quasi-bisdisphenoids (cC, orange). Note that the topologies ncb , bcu and nbo all possess the cubic symmetry (black lines represent the unit cell). Full size image As is in the case of other prototypes, the solvent-accessible void of the ncb framework is dependent on the length of each ligand. The calculated crystal densities and pore volumes for Ia - Vd are 0.39–1.06 g cm −3 and 0.49–2.04 cm 3 g −1 , respectively ( Fig. 3a ). With N 2 as a probe, the calculated accessible surface areas of the isoreticular frameworks vary from 970 to 4,760 m 2 g −1 ( Fig. 3b ) [52] . More interestingly, changing the ratio of the lengths between pyridylcarboxylate and dicarboxylate can anisotropically modulate the pore size/shape ( Fig. 3c ; Supplementary Figs S33–S45 ; Supplementary Table S5 ). The shape of cA is basically maintained as a regular tetrahedron, and its size is only determined by the dicarboxylate length, which has a diameter of 7.8, 9.4, 11.2 and 13.0 Å for bdc 2– , ndc 2– , bpdc 2– and edba 2– , respectively. In contrast, the shape of cB can be tuned by d r or the ratio of lengths of the two linkers. When d r ≈1 (for example, IIIb ), the shape of cB is tetrahedral (similar to that of cA). Otherwise, cB becomes elongated ( d r >1, for example, IIIb ) or flattened ( d r <1, for example, IIIc ). It should be noted that isoreticular PCPs with changeable pore shapes are still rarely encountered in the literature [42] , [43] , [44] , [45] , [46] . As cC is mainly composed of pyridylcarboxylate edges, its shape is basically unchanged, and its size is mainly determined by the pyridylcarboxylate length, which is about 7.4, 10, 12, 14 and 17 Å for ina − , pyac − , pba − , pvba − and pbpa − , respectively. Furthermore, such a systematic modulation can finally alter the relative volume ratio between the channel and the cavities of each framework ( Fig. 3d ; Supplementary Table S5 ). For instance, the relative channel/cavity volume ratios are 2.31, 1.72 and 1.51 for IIIa , IIIb and IIIc , respectively, which combine the same pyridylcarboxylate pba − with longer dicarboxylates bdc 2– , ndc 2– and bpdc 2– . 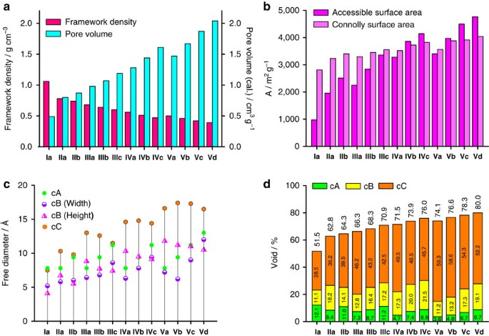Figure 3: Systematic modulation of pore metrics. (a) Framework densities and pore volumes. (b) Accessible and Connolly surface areas. (c) Pore sizes of three types of cavities. (d) Total and individual percentages of volume of the three types of cavities. Figure 3: Systematic modulation of pore metrics. ( a ) Framework densities and pore volumes. ( b ) Accessible and Connolly surface areas. ( c ) Pore sizes of three types of cavities. ( d ) Total and individual percentages of volume of the three types of cavities. Full size image A comparison of determined crystal structures with the corresponding predicted ncb network models (with different d r values) can provide a better understanding of how the molecular building blocks adjust their shapes to fit the node geometries. Several parameters were used to evaluate the geometries of the SBUs and the ligands, as well as the connection between them, which include the deviation angle of the coordinated nitrogen atom from the triangular Ni 3 plane ( κ ′), the angle between the pyridyl group and the corresponding N–Ni bond ( κ ″), the included angles of two adjacent carboxylate groups between two pyridylcarboxylates ( φ ′) and between two dicarboxylates ( ω ′), and the bending degrees of the pyridylcarboxylate ( δ 1 ) and dicarboxylate ( δ 2 ), defined as the ratio of arced height over chord length of the ligands ( Fig. 4 ). 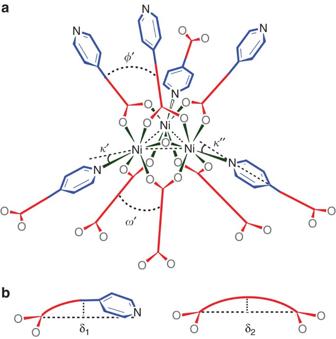Figure 4: Schematic illustration of the distortion of the molecular building blocks in the isoreticular frameworks. (a) Distortions of the trinuclear SBU can be described by three parameters, that is,κ′for the deviation angle of coordinated nitrogen atom from the triangular Ni3plane (κ′=0° for the non-distorted structure),φ′for the included angle of two adjacent carboxylate groups between two pyridylcarboxylates (φ′=70° for the non-distorted structure), andω′for the included angle of two adjacent carboxylate groups between two dicarboxylates (ω″=70° for the non-distorted structure). The distorted connection between the trinuclear SBU and the ligands can be evaluated by the included angle between the pyridyl group and corresponding N–Ni bond (κ″). (b) Distortions of the organic ligands are defined as the ratio of arced height over chord length of the ligands, usingδ1for the pyridylcarboxylate andδ2for the dicarboxylate (except the pyridyl rings, the aromatic backbones are simplified as solid lines for clarity). Figure 4: Schematic illustration of the distortion of the molecular building blocks in the isoreticular frameworks. ( a ) Distortions of the trinuclear SBU can be described by three parameters, that is, κ′ for the deviation angle of coordinated nitrogen atom from the triangular Ni 3 plane ( κ′ =0° for the non-distorted structure), φ′ for the included angle of two adjacent carboxylate groups between two pyridylcarboxylates ( φ′ =70° for the non-distorted structure), and ω′ for the included angle of two adjacent carboxylate groups between two dicarboxylates ( ω″ =70° for the non-distorted structure). The distorted connection between the trinuclear SBU and the ligands can be evaluated by the included angle between the pyridyl group and corresponding N–Ni bond ( κ″ ). ( b ) Distortions of the organic ligands are defined as the ratio of arced height over chord length of the ligands, using δ 1 for the pyridylcarboxylate and δ 2 for the dicarboxylate (except the pyridyl rings, the aromatic backbones are simplified as solid lines for clarity). Full size image As shown in Table 1 , the κ ′ angles are basically very small in contrast to the corresponding κ angles, illustrating the binding rigidity of the SBUs' equatorial planes. With a relatively short and rigid pyridylcarboxylate pba − , κ ″ (2.2, 4.8 and 9.3° for IIIa , IIIb and IIIc , respectively) increases along with increasing κ (6.9, 12.2 and 17.5° for IIIa , IIIb and IIIc , respectively), suggesting that the structure adjustment or compensation starts by bending the pyridyl rings from the Ni–N bond directions, with the pyridyl N atom as the knee, which should be energetically unstable compared with a linear pyridyl-metal coordination (that is, κ ″=0°). The residual required κ ( κ > κ ′+ κ ″) is finally achieved by bending the pba − backbone (2.3, 4.3 and 5.4%). For the longer and more flexible pvba − , κ ″ in IVa , IVb and IVc (2.0°, 1.4° and 3.2°, respectively) basically remains unaltered albeit κ is 3.5°, 7.8° and 12.5°, respectively. Obviously, the required distortions are mainly provided by the inherently bent pvba − ( δ 1 =9.0, 11.6 and 8.0%). Table 1 Comparison of framework distortion with thermal stability. Full size table With an even longer but relatively rigid pbpa − , the situation is more complicated. The observed κ ′ (1.4°), κ ′, (0.8°) and δ (5.4%) are reasonable for Vc . However, κ ′ (2.9° and 1.4°) and κ ″ (1.9° and 4.7°) exceed the κ (0.9° and 4.7°) for Va and Vb , respectively. Moreover, the observed φ ′ angle (24.1°) for Va is not located between the required φ angle (35.1°) and the ideal value of 70°. A detailed inspection of the crystal structure reveals that the SBU is now distorted from C 3 v to C 3 symmetry by twisting the carboxylate groups of the pbpa − ligands, which avoids the steric hindrance required by the extremely small φ . These significant distortions are compensated for by changing in the other segments of the whole network, that is, κ ′ and κ ″. With larger φ angles, the carboxylate groups of pyridylcarboxylates are less distorted in Vb and almost not distorted in Vc . The small φ in IVa could be compensated for by the flexible pvba − . As the capped binding sites of SBU possess specifically pointing directions, the linkers should possess enough length or flexibility to compensate for the required κ, although the steric hindrance between the adjacent carboxylate groups requires them to twist in a skew-coordination manner to adopt the extremely small φ angles. Therefore, shorter and/or less flexible linkers can hardly fulfill the required bending or avoid the steric hindrance in forming the ncb frameworks. The above discussions may be useful for understanding the difficulty in the synthesis of Ia ( κ ′+ κ ″=16.7°), IIb ( κ ′+ κ ″=12.9°), IIIc ( κ ′+ κ ″=9.3°), IVc ( δ 1 =8.0%) and Va ( φ ′=24.9°). Thermal stabilities Although the thermal stability of PCPs is usually ascribed to the porosity and robustness of the coordination bonds, the SBU and the organic ligand, the structural stability of the underlying prototype or the inner tension of the framework has been rarely considered. In this context, the isoreticular frameworks obtained in this work represent an inherently tensile system for studying the influence of porosity and framework distortion on the thermal stability. Although thermogravimetric analyses showed that all the isoreticular frameworks similarly decomposed above 350 °C ( Supplementary Fig. S46 ), variable-temperature powder X-ray diffraction ( Supplementary Figs S47–S58 ) studies indicated that their critical temperatures of framework collapse ( T c ) are very different from each other, and also are obviously lower than 350 °C ( Table 1 ). Considering that common isoreticular PCPs usually collapse at similar temperatures [16] , the above observation implies that the isoreticular ncb frameworks studied here possess notable and different degrees of inner tensions. Although the T c values of the studied ncb frameworks basically decrease as the porosity increases, they could not be explained solely by the voids or pore volumes of the corresponding crystal structures. Alternatively, the node geometry may also be an influencing factor. Taking IIIa (void=66.3%, κ ″=2.2°, T c =300 °C), IIIb (void=68.2%, κ″=4.8°, T c =240 °C) and IIIc (void=70.9%, κ ″=9.3°, T c =210 °C) as an example, the void just grows slightly, but T c steeply decreases, which could be explained by the fast-growing κ ″. The importance of the framework distortion may be greater than that of porosity, which can be illustrated by comparison between IVa (void=71.5%, κ ″=2.0°, T c =250 °C) and IIIc (void=70.9%, κ ″=9.3°, T c =210 °C), and also between Vb (void=76.6%, κ ″=4.7°, T c =160 °C) and Vc (void=78.3%, κ ″=0.8°, T c =180 °C). Adsorption properties Porous properties of IIIa , IIIb and IIIc were characterized by N 2 , CO 2 and H 2 sorption measurements. As seen from their crystal structures, the three compounds possess not only gradually increasing total pore volumes/sizes very similar to other reported isoreticular PCPs, but also very different channel-cavity characteristics (pore sizes/shapes are very similar for nbo channels, but very different for bcu cavities). These characteristics would be useful for revealing the structural modulation effect of the ternary prototype ncb . For comparison, the same measurements were also performed for Ia with a significantly smaller pore size. As shown in Supplementary Figures S59 and S60 , the four isoreticular frameworks can be readily activated for gas sorption measurements. N 2 isotherms of IIIa , IIIb and IIIc revealed apparent Langmuir surface areas of 2,681, 2,706 and 2,841 m 2 g −1 , Brunauer–Emmett–Teller surface areas of 2,525, 2,610 and 2,738 m 2 g −1 , and pore volumes (Dubinin–Astakhov) of 0.95, 0.96 and 1.04 cm 3 g −1 , respectively, being similar to those predicted from their crystal structures ( Fig. 5a ). Low-pressure H 2 adsorption isotherms for IIIa , IIIb and IIIc showed similar gravimetric uptakes of ca. 1.7 wt% ( Fig. 5b ), but decreasing volumetric uptakes of 11.5, 10.5 and 9.8 g l −1 , respectively, at 1 bar and 77 K ( Fig. 5c ), consistent with their similar surface areas and pore volumes, as well as different framework densities. High-pressure sorption measurements showed very high gravimetric ( Fig. 5d ) and volumetric ( Supplementary Fig. S61 ) H 2 uptakes for IIIa , IIIb and IIIc at 77 K and 50 bar. However, all three isotherms have not reached saturation at the highest measured pressures, which can be ascribed to the inert pore surfaces (there are no active sites such as a coordinatively unsaturated metal centre) and large pore sizes. Nevertheless, the excess and absolute H 2 uptakes follow IIIa > IIIb > IIIc , indicating that the host–guest interactions or confinement effects are stronger for a smaller pore size [53] . In comparison with IIIa – IIIc , Ia possesses much smaller pore sizes and have a substantially lower surface area (1,019 and 880 m 2 g −1 for Langmuir and Brunauer–Emmett–Teller, respectively), a pore volume (0.36 cm 3 g −1 ) and a H 2 -uptake capacity, but has a stronger adsorption at low pressures. The above discussions about host–guest interactions were confirmed by the H 2 adsorption enthalpies calculated by isotherms measured at 77 and 87 K ( Supplementary Fig. S62 ). The H 2 adsorption enthalpy at zero coverage is ca. 8.0 kJ mol −1 for Ia , being similar to other ultramicroporous frameworks. In contrast, the large-pore frameworks IIIa , IIIb and IIIc possess lower enthalpies around 4.5–5.5 kJ mol −1 ( Fig. 5e ). 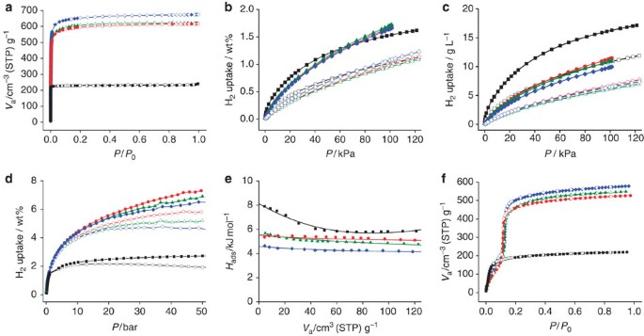Figure 5: Gas sorption properties. (a) N2sorption adsorption (filled) and desorption (open) isotherms measured at 77 K, (b) gravimetric H2uptakes measured at 77 K (filled) and 87 K (open) up to 120 kPa, (c) volumetric H2uptakes measured at 77 K (filled) and 87 K (open) up to 120 kPa, (d) excess (open) and absolute (filled) H2uptakes measured at 77 K up to 50 bar, (e) coverage-dependent H2adsorption enthalpies calculated from the low-pressure isotherms measured at 77 and 87 K by the virial fitting method (lines) and Clausius–Claperyron equation (symbols), and (f) CO2adsorption (filled) and desorption (open) isotherms measured at 195 K forIa(black),IIIa(red),IIIb(green) andIIIc(blue). Figure 5: Gas sorption properties. ( a ) N 2 sorption adsorption (filled) and desorption (open) isotherms measured at 77 K, ( b ) gravimetric H 2 uptakes measured at 77 K (filled) and 87 K (open) up to 120 kPa, ( c ) volumetric H 2 uptakes measured at 77 K (filled) and 87 K (open) up to 120 kPa, ( d ) excess (open) and absolute (filled) H 2 uptakes measured at 77 K up to 50 bar, ( e ) coverage-dependent H 2 adsorption enthalpies calculated from the low-pressure isotherms measured at 77 and 87 K by the virial fitting method (lines) and Clausius–Claperyron equation (symbols), and ( f ) CO 2 adsorption (filled) and desorption (open) isotherms measured at 195 K for Ia (black), IIIa (red), IIIb (green) and IIIc (blue). Full size image The CO 2 sorption isotherms of IIIa , IIIb and IIIc showed obvious two-step features ( Fig. 5f ). Careful examination of the CO 2 isotherm of Ia also revealed an unobvious step at low relative pressure ( Supplementary Fig. S63 ). Previously, a gating mechanism, that is, before the step adsorption occurred only in the nbo channel, and after the step adsorption occurred in both the nbo channel and bcu cavities, was proposed to explain the two-step CO 2 isotherm shape for IIIb , because the small aperture (aBC) between the nbo channel and bcu cavity may block the diffusion of CO 2 , which was well supported by the Langmuir surface areas of the two steps [48] . Obviously, the gating mechanism cannot simultaneously explain the four CO 2 isotherms as shown in Figure 5f and Supplementary Figure S63 , because the onset pressure of the step is lower for the smaller gate size. On the basis of the structural relationships of the measured isoreticular frameworks, the four CO 2 isotherms can be elucidated by a capillary condensation mechanism. The small slopes before the steps are related to the weak host–guest interaction. The onset pressure of the step (capillary condensation starts) is lower for smaller pores. To examine the pore size/shape effect on guest diffusion, CO 2 adsorption kinetic data were measured, which can be fitted well by a double-exponential model ( Supplementary Figs S64–S67 ). In other words, the CO 2 diffusion in the hierarchical pore systems could be divided into a fast component within the large nbo channel (determined by aCC) and a slow one through the small entrances of the bcu cavities (determined by aBC) [54] . As shown in Supplementary Figures S68–S71 , the small aBC apertures in IIIa and IIIb comparable to the size of CO 2 exhibit an obvious restriction on the diffusion into the bcu cavities, which may be overwhelmed by increasing the pressure. In contrast, IIIc with obviously larger aBC apertures has no such effect, and the main restriction should likely arise from steric hindrance of the adsorbed CO 2 molecules. In this context, the isoreticular ncb frameworks with well-controlled hierarchical biporous structures can demonstrate systematical modulation on not only the surface area, pore volume and sorption affinity, but also guest diffusion kinetics. The simple, highly symmetric ncb topology represents a novel ternary network prototype, in which the pore size/shape and the cavity/channel void ratio can be altered by changing the two kinds of linkers. Unlike other well-studied prototypes, even the most suitable molecular building blocks still deviate obviously from the network geometry of ncb , representing a challenge for the rational design and construction of this unique structure. Using a geometry analysis approach, we showed that the difficulty of construction of the ncb -type frameworks can be evaluated simply by the ratio of the lengths of the two kinds of ligands. A new series of highly porous, isoreticular frameworks have been constructed, which illustrate systematic adjustment of pore size and anisotropic modulation of pore shapes, as well as the influence of the ligand–length ratio on the geometry of the molecular building blocks and the framework stabilities. Although computer modelling (for example, quantum/molecular mechanics) is very powerful for predicting the properties of molecules and crystalline networks, the geometry analysis approach is simple, fast, facile and efficient for even very complicated systems (containing a large number of atoms and/or transition metal, especially open-shell ones). Also, the geometry analysis results of isostructural structures with different number and type of atoms can be directly compared. Considering that numerous topologies have been known, many of which have similar complexity to ncb , the geometry analysis method or mathematical idea may be applied for other prototypes and enlighten crystal design and targeted assembly of new PCPs. Materials The ligands H 2 tpdc, Hpba, Hpvba and Hpbpa were synthesized according to the literature ( Supplementary Methods ). Other reagents were commercially available and used without further purification. Preparation of isoreticular frameworks A methanol (2.0 ml) solution of Ni(NO 3 ) 2 .6H 2 O was added into an amide solution (22 ml) of pyridylcarboxylic acid, dicarboxylic acid and NaOH (or 40% tetrabutylammonium hydroxide methanol solution). The mixture was heated at 65 °C and stirred for 1 h, and then sealed in a 50-ml Teflon-lined stainless steel vessel, which was heated to 120–160 °C for 72 h. Upon cooling down to room temperature at a rate of 5 °C h −1 , solid products were isolated by filtration or centrifuge, which were identified by single-crystal X-ray diffraction and/or powder X-ray diffraction (PXRD) analyses. After many trials, 13 targeted compounds have been successfully isolated, whose chemical formulae and purity were confirmed by PXRD ( Supplementary Figs S17–S28 ), elemental analysis (EA), Fourier-transform infrared spectra ( Supplementary Methods ), magnetic susceptibility measurement ( Supplementary Figs S30–S32 and Supplementary Methods ) and thermogravimetric analysis ( Supplementary Fig. S46 ). [Ni 3 (μ 3 -OH)(ina) 3 (bdc) 1.5 ]·2.5DMA·CH 3 OH ( Ia ) was prepared by mixing Ni(NO 3 ) 2 .6H 2 O (1,740 mg, 6.0 mmol), Hina (738 mg, 6.0 mmol), H 2 bdc (498 mg, 3.0 mmol) and NaOH (560 mg, 14.0 mmol) in N , N ′-dimethylacetamide (DMA) at 160 °C (yield 650 mg, ca. 30%). EA calculated (%) for C 41 H 45.5 N 5.5 O 16.5 Ni 3 : C 46.66, H 4.35, N 7.30; found: C 46.46, H 4.50, N 7.36. [Ni 3 (μ 3 -OH)(pyac) 3 (bdc) 1.5 ]·5.5DMF·5.5H 2 O ( IIa ) was prepared by mixing Ni(NO 3 ) 2 .6H 2 O (435 mg, 1.5 mmol), Hpyac (220 mg, 1.5 mmol), H 2 bdc (125 mg, 0.75 mmol) and tetrabutylammonium hydroxide (2.5 ml, 3.5 mmol) in N , N ′-dimethylformide (DMF) at 140 °C (yield 120 mg, ca. 20%, poor reproducibility). EA calculated (%) for C 52.5 H 74.5 N 8.5 O 24 Ni 3 : C 45.54, H 5.42, N 8.60; found: C 45.23, H 5.01, N 8.78. [Ni 3 (μ 3 -OH)(pyac) 3 (ndc) 1.5 ]·6DMF·6H 2 O ( IIb ) was prepared by mixing Ni(NO 3 ) 2 .6H 2 O (435 mg, 1.5 mmol), Hpyac (220 mg, 1.5 mmol), H 2 ndc (162 mg, 0.75 mmol) and tetrabutylammonium hydroxide (2.5 ml, 3.5 mmol) in DMF at 140 °C (yield 230 mg, ca. 30%). EA calculated (%) for C 60 H 82 N 9 O 25 Ni 3 : C 47.87, H 5.49, N 8.37; found: C 47.00, H 6.03, N 8.94. [Ni 3 (μ 3 -OH)(pba) 3 (bdc) 1.5 ]·8DMA·2CH 3 OH·4H 2 O ( IIIa ) was prepared by mixing Ni(NO 3 ) 2 .6H 2 O (870 mg, 3.0 mmol), Hpba (600 mg, 3 mmol), H 2 bdc (250 mg, 1.5 mmol) and NaOH (280 mg, 7.0 mmol) in DMA at 160 °C (yield 1,300 mg, ca. 70%). EA calculated (%) for C 82 H 119 N 11 O 27 Ni 3 : C 52.75, H 6.42, N 8.25; found: C 52.38, H 6.48, N 8.66. [Ni 3 (μ 3 -OH)(pba) 3 (ndc) 1.5 ]·10.5DMA·2CH 3 OH·2H 2 O ( IIIb ) was prepared by mixing Ni(NO 3 ) 2 .6H 2 O (870 mg, 3.0 mmol), Hpba (600 mg, 3 mmol), H 2 ndc (330 mg, 1.5 mmol) and NaOH (280 mg, 7.0 mmol) in DMA at 160 °C (yield 1,400 mg, ca. 65%). EA calculated (%) for C 98 H 140.5 N 13.5 O 27.5 Ni 3 : C 55.42, H 6.67, N 8.90; found: C 54.13, H 6.70, N 9.08. [Ni 3 (μ 3 -OH)(pba) 3 (bpdc) 1.5 ]·11.5DMA·0.5CH 3 OH·7H 2 O ( IIIc ) was prepared by mixing Ni(NO 3 ) 2 .6H 2 O (870 mg, 3.0 mmol), Hpba (600 mg, 3 mmol), H 2 bpdc (380 mg, 1.5 mmol) and NaOH (280 mg, 7.0 mmol) in DMA at 160 °C (yield 1,000 mg, ca. 45%, poor reproducibility). EA calculated (%) for C 103.5 H 156.5 N 14.5 O 32 Ni 3 : C 54.24, H 6.88, N 8.86; found: C 53.98, H 7.06, N 9.00. [Ni 3 (μ 3 -OH)(pvba) 3 (bdc) 1.5 ]11.5DMA11H 2 O ( IVa ) was prepared by mixing Ni(NO 3 ) 2 .6H 2 O (870 mg, 3.0 mmol), Hpvba (670 mg, 3 mmol), H 2 bdc (250 mg, 1.5 mmol) and NaOH (280 mg, 7.0 mmol) in DMA at 160 °C (yield 900 mg, ca. 40%). EA calculated (%) for C 100 H 162.5 N 14.5 O 35.5 Ni 3 : C 51.95, H 7.08, N 8.78; found: C 51.79, H 6.92, N 8.98. [Ni 3 (μ 3 -OH)(pvba) 3 (ndc) 1.5 ]15DMA·10H 2 O ( IVb ) was prepared by mixing Ni(NO 3 ) 2 .6H 2 O (870 mg, 3.0 mmol), Hpvba (670 mg, 3 mmol), H 2 ndc (33 mg, 0.15 mmol) and NaOH (280 mg, 7.0 mmol) in DMA at 160 °C (yield 1,600 mg, ca. 60%). EA calculated (%) for C 120 H 195 N 18 O 38 Ni 3 : C 53.90, H 7.35, N 9.43; found: C 53.42, H 7.38, N 9.57. [Ni 3 (μ 3 -OH)(pvba) 3 (bpdc) 1.5 ]·16.5DMA·CH 3 OH·10.5H 2 O ( IVc ) was prepared by mixing Ni(NO 3 ) 2 .6H 2 O (870 mg, 3.0 mmol), Hpvba (670 mg, 3 mmol), H 2 bpdc (380 mg, 1.5 mmol) and NaOH (280 mg, 7.0 mmol) in DMA at 160 °C (yield 280 mg, ca. 10%). EA calculated (%) for C 130 H 216.5 N 19.5 O 41 Ni 3 : C 54.12, H 7.56, N 9.47; found: C 53.14, H 7.22, N 9.48. [Ni 3 (μ 3 -OH)(pbpa) 3 (bdc) 1.5 ]12DMA7CH 3 OH ( Va ) was prepared by mixing Ni(NO 3 ) 2 .6H 2 O (435 mg, 1.5 mmol), Hpbpa (415 mg, 1.5 mmol), H 2 bdc (125 mg, 0.75 mmol) and tetrabutylammonium hydroxide (2.5 ml, 3.5 mmol) in DMA at 150 °C (yield 140 mg, ca. 10%). EA calculated (%) for C 121 H 179 N 15 O 32 Ni 3 : C 57.40, H 7.13, N 8.30; found: C 56.80, H 8.24, N 8.43. [Ni 3 (μ 3 -OH)(pbpa) 3 (ndc) 1.5 ]15DMA20H 2 O ( Vb ) was prepared by mixing Ni(NO 3 ) 2 .6H 2 O (435 mg, 1.5 mmol), Hpbpa (415 mg, 1.5 mmol), H 2 ndc (165 mg, 0.75 mmol) and tetrabutylammonium hydroxide (2.5 ml, 3.5 mmol) in DMA at 150 °C (yield 230 mg, ca. 15%). EA calculated (%) for C 132 H 221 N 18 O 48 Ni 3 : C 52.77, H 7.41, N 8.39; found: C 52.44, H 6.95, N 8.72. [Ni 3 (μ 3 -OH)(pbpa) 3 (bpdc) 1.5 ]22DMA28H 2 O ( Vc ) was prepared by mixing Ni(NO 3 ) 2 .6H 2 O (435 mg, 1.5 mmol), Hpbpa (415 mg, 1.5 mmol), H 2 bpdc (190 mg, 0.75 mmol) and tetrabutylammonium hydroxide (2.5 ml, 3.5 mmol) in DMA at 150 °C (yield 760 mg, ca. 40%). EA calculated (%) for C 163 H 303 N 25 O 63 Ni 3 : C 51.56, H 8.04, N 9.22; found: C 51.57, H 7.56, N 9.21. [Ni 3 (μ 3 -OH)(pba) 3 (edba) 1.5 ]· x G ( Vd ) was obtained by mixing Ni(NO 3 ) 2 .6H 2 O (87 mg, 0.3 mmol), Hpbpa (83 mg, 0.3 mmol), H 2 edba (40 mg, 0.15 mmol) and tetrabutylammonium hydroxide (2.5 ml, 3.5 mmol) in DMA at 150 °C. Only a few crystals have been isolated for single-crystal diffraction study and the reproducibility is very poor. The unsuccessful combinations were retried with modified synthetic conditions (different solvents or mixed solvents, stoichiometric ratios of reactants, synthetic temperature and time, and so on); however, only some unidentified microcrystalline products or amorphous floccules were obtained ( Supplementary Table S2 and Supplementary Fig. S29 ). Measurements Elemental analyses were performed using the Vario EL element analyzer with as-synthesized sample. Thermogravimetric analyses were carried out using a TA Instruments Q50 Thermogravimetric Analyzer under N 2 at the rate of 5 °C min −1 . PXRD patterns were recorded on a Bruker D8-Advance diffractometer using Cu Kα radiation and LynxEye detector. Variable-temperature PXRD analyses were facilitated with an Anton Paar TTK-450 sample stage under N 2 flow. The temperature was increased at the rate of 0.1 °C s −1 , and kept for 15 min before measurement at each targeted temperature. Magnetic property measurements were carried on a Quantum Design SQUID magnetometer MPMS XL-7 using degassed samples. X-ray single-crystal structure analyses Diffraction data were collected on a Bruker APEX CCD Diffractometer with graphite-monochromated Mo Kα radiation or an Oxford Gemini S Ultra CCD diffractometer using mirror-monochromated Cu Kα radiation. The crystal structures were solved through Patterson methods and developed by difference Fourier techniques using the SHELXTL and Olex 2 software packages. Structures Ia , IIIa , IIIc , Va and Vc were well solved in the I -43 m space group, because their ligands obey the symmetry requirement of the maximum-symmetry form of ncb net; that is, E 1 (pyridylcarboxylate) possesses m symmetry and E 2 (dicarboxylate) possesses mm 2 symmetry. The absence of the mm 2 symmetry of dicarboxylates may lead to lower symmetry structures I 23 ( IIIb and Vb ). The absence of the m symmetry of the pyridylcarboxylates can lead to another lower-symmetry structure of P -43 n ( IIb ). Solving these structures in I -43 m resulted in symmetry-imposed disorder of the ligands. In some cases, low-symmetry ligands may be statistically disordered in I 23, P -43 n and I -43 m . Therefore, their structures were solved in the high-symmetry space group I -43 m ( IIa , IVa , IVb , IVc and Vd ). As some phenyl rings are disordered, appropriate restraints were applied in the refinements. Hydrogen atoms were generated geometrically and refined using a riding model. As the very disordered solvent molecules could not be modelled, PLATON/SQUEEZE procedures were used to remove the contribution of reflection by the guest solvent molecules. Crystallographic data for Ia , IIa , IIb , IIIa , IIIb , IIIc , IVa , IVb , IVc , Va , Vb , Vc and Vd have been deposited in the Cambridge Crystallographic Data Center under deposition numbers CCDC 856758–856770 ( Supplementary Data 1 ). Sorption measurements and analyses As-synthesized samples were immersed in dichloromethane for 3–5 days, during which dichloromethane was refreshed three times a day. After that, the samples were washed by acetone for several times, then filtered and quickly transferred to the sample cells for sorption measurements. Thermogravimetric analysis and PXRD were applied to confirm the complete solvent exchange and retention of crystallinity ( Supplementary Figs S59 and S60 ). Low-pressure gas sorption experiments (up to 120 kPa) were carried out on a Micromeritics ASAP 2020 M Physisorption Analyzer. Ultrahigh-purity-grade (purity >99.999%) N 2 , H 2 , CO 2 and He gases were used in all adsorption measurements. High-pressure H 2 sorption experiments (0~50 bar) were carried out on a BELSORP-HP volumetric adsorption apparatus. Temperatures were maintained by liquid nitrogen, liquid argon and dry ice-acetone baths. The coverage-dependent adsorption enthalpies (isosteric heat, Q st ) of H 2 were calculated from the sorption data measured at 77 and 87 K by the virial fitting method and the Clausius–Claperyron equation. Kinetic data for CO 2 adsorption at 195 K were collected simultaneously with the isotherms by the rate of adsorption function. How to cite this article: Zhang, Y.-B. et al . Geometry analysis and systematic synthesis of highly porous isoreticular frameworks with a unique topology. Nat. Commun. 3:642 doi: 10.1038/ncomms1654 (2012).